Tetrasaccharide iteration synthesis of a heparin-like dodecasaccharide and radiolabelling forin vivotissue distribution studies Heparin-like oligosaccharides mediate numerous important biological interactions, of which many are implicated in various diseases. Synthetic improvements are central to the development of such oligosaccharides as therapeutics and, in addition, there are no methods to elucidate the pharmacokinetics of structurally defined heparin-like oligosaccharides. Here we report an efficient two-cycle [4+4+4] tetrasaccharide-iteration-based approach for rapid chemical synthesis of a structurally defined heparin-related dodecasaccharide, combined with the incorporation of a latent aldehyde tag, unmasked in the final step of chemical synthesis, providing a generic end group for labelling/conjugation. We exploit this latent aldehyde tag for 3 H radiolabelling to provide the first example of this kind of agent for monitoring in vivo tissue distribution and in vivo stability of a biologically active, structurally defined heparin related dodecasaccharide. Such studies are critical for the development of related saccharide therapeutics, and the data here establish that a biologically active, synthetic, heparin-like dodecasaccharide provides good organ distribution, and serum lifetimes relevant to developing future oligosaccharide therapeutics. Heparin and heparan sulphate (H/HS) are ubiquitous linear polysulphated oligosaccharides of the glycosaminoglycan (GAG) family, comprising a repeating disaccharide unit. Because of its structural heterogeneity, H/HS is crucially involved in regulating a myriad of cell signalling pathways through modulation of interactions between cytokines and their receptors. This is typified through its involvement in the mediation of fibroblast growth factor (FGF)-regulated cell phenotypes, such as proliferation, adhesion, motility and angiogenesis [1] , [2] , [3] , [4] , [5] , [6] , [7] . Although methods for the isolation of natural H/HS samples from biochemical degradation processes are well-established [8] , [9] , synthetic access to structurally defined H/HS mimetics has also received very significant attention [10] , [11] , [12] , [13] , [14] , [15] , [16] , [17] , [18] , [19] , [20] , [21] , [22] , [23] , [24] , [25] , [26] , [27] , [28] , [29] , [30] , [31] , [32] , [33] , [34] , [35] , [36] . Synthetic access is essential to provide structurally defined H/HS oligosaccharide sequences to interrogate the chemical biology of H/HS-mediated processes, a better understanding of which also offers the potential to aid development of new disease treatments [37] , [38] , [39] , [40] , [41] . The potential development of such oligosaccharides as therapeutics is also dependent on developing tools to determine the pharmacokinetics, distribution and organ availability of these synthetic species. To date, the limitations of synthetic access to suitable tools has precluded such developments for bioactive lead oligosaccharide structures. This presents the need to develop an efficient procedure for the synthesis of longer bioactive heparin-like oligosaccharides, which also provide efficient access to derivatization/conjugation of structurally defined, biologically significant synthetic H/HS sequences [42] , [43] , [44] , [45] . Our previous in vitro and in vivo anti-angiogenic assessments of size-fractionated digests [46] , [47] , [48] , [49] , [50] , [51] and subsequent evaluation of a matrix of structurally defined synthetic oligosaccharides [52] indicated that longer [GlcNS-IdoA2S]-containing species were more effective inhibitors of FGF2, and identified the methyl glycoside analogue of dodecasaccharide 1 ([GlcNS-IdoA2S] 6 -OMe) as the optimum lead FGF2 and vascular endothelial growth factor antagonist [52] ( ex vivo evaluation of the synthetic dodecasaccharide [GlcNS-IdoA2S] 6 -OMe confirmed that at biologically active concentrations inhibiting FGF signalling, there was no statistically significant impact on anticoagulation, an important feature required for potential development of therapeutic synthetic saccharides of this type). Here we report a powerful addition to the field of synthetic heparanoid chemistry, which demonstrates an efficient chemical synthesis of this structurally defined [GlcNS-IdoA2S] 6 heparin-like lead dodecasaccharide 1 , bearing a terminal latent aldehyde tag (LAT), in just two iterative cycles and four steps from a precursor tetrasaccharide. Concomitant LAT release in a final-step modification of the oligosaccharide is applied to 3 H radiolabelling of dodecasaccharide 1 with minimal structural impact. This demonstrates the viability of the approach for rapid, iterative synthetic access to large oligosaccharides on useful scales, which are suitable for biological conjugations and labelling. The tritium radiolabelled analogue 1 , which provides a new tool to determine the pharmacokinetics of the synthetic oligosaccharide and establish the organ distribution and in vivo lifetime of the lead dodecasaccharide 1 , critical factors for the potential development of HS oligosaccharide therapeutics. Strategy and end labelling The end modification of oligosaccharides (via ring opening of the terminal acetal unit, for example, for attaching fluorophores) is an established method for labelling native heparin and related GAGs to facilitate their separation or analysis [53] , [54] . A number of examples have also employed amide derivatization of the uronic carboxylates to introduce fluorescent or spin labels, or to attach conjugates [55] , [56] . There are also a range of uses of modified O -glycosides recently employed for conjugation, surface and nanoparticle/dendrimer attachments [42] , [43] , [44] , [45] , including applications of click chemistry, in particular the Huisgen reaction. However, an alternative approach was needed to ensure compatibility with the deprotection/labelling conditions during synthesis and introducing minimal change to the polarity/functional groups of the oligosaccharide. Thus, a 1,2-diol moiety at the reducing end was incorporated as an LAT. Having an additional O4-sulphate at the non-reducing end of the deprotected dodecasaccharide would allow complete selectivity in a final-stage periodate-mediated cleavage of the LAT to liberate a reactive aldehyde tag (RAT) directly on the final oligosaccharide, thus allowing facile reductive labelling or facilitating other conjugations. Our approach was to develop this LAT incorporation concurrently with the aforementioned tetrasaccharide iteration strategy ( Fig. 1 ). 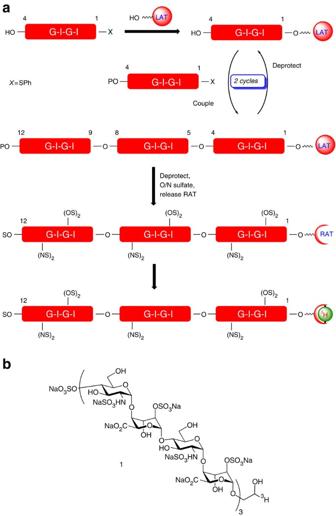Figure 1: Strategy for synthesis of end-labelled dodecassacharide. (a) Iterative [4+4+4] oligosaccharide synthesis strategy with final step RAT release and labelling. G, Glucosamine unit; I, iduronate unit; P, trichloroacetyl; S, SO3Na; LAT, latent aldehyde tag; RAT, reactive aldehyde tag. (b) Structure of radiolabelled dodecasaccharide. Figure 1: Strategy for synthesis of end-labelled dodecassacharide. ( a ) Iterative [4+4+4] oligosaccharide synthesis strategy with final step RAT release and labelling. G, Glucosamine unit; I, iduronate unit; P, trichloroacetyl; S, SO 3 Na; LAT, latent aldehyde tag; RAT, reactive aldehyde tag. ( b ) Structure of radiolabelled dodecasaccharide. Full size image Synthesis of tetrasaccharide building blocks The synthetic strategy envisaged using one precursor disaccharide building block, 2 , to provide a single tetrasaccharide unit, 7 , which would function both as an iterative donor (as its O4-trichloroacetyl derivative 8 ) and as an immediate precursor to an LAT-bearing tetrasaccharide, serving as the initial acceptor tetrasaccharide. Disaccharide 2 was prepared as reported previously, exploiting our scalable iduronate thioglycoside acceptor capabilities for constructing such reagents [57] , [58] , and is a reverse of the common IdoA-GlcN disaccharide repeat unit seen in several previous heparin-related syntheses [10] , [11] , [12] , [13] , [14] , [15] , [16] , [17] , [18] , [19] , [20] , [21] , [22] , [23] , [24] , [25] , [26] , [27] , [28] , [29] , [30] , [31] , [32] , [33] , [34] , [35] , [36] . Disaccharide 2 was divergently elaborated into trichloroacetimidate donor 4 (see Supplementary Figs S5–S12 ) via free sugar disaccharide 3 (see Supplementary Figs S1–S4 ) and acceptor 5, with these two building blocks then efficiently coupled to afford tetrasaccharide 6 ( Fig. 2 ; see Supplementary Figs S13–S17 ). Deprotection at the non-reducing end terminus of 6 then provided the required tetrasaccharide 7 (see Supplementary Figs S18–S22 ), which was also protected as its O4-TCA derivative 8 (see Supplementary Figs S23–S31 ), thereby providing two potential tetrasaccharide donor modules ( 6 and 8 ), differing only in their non-reducing terminal O4-protecting group. 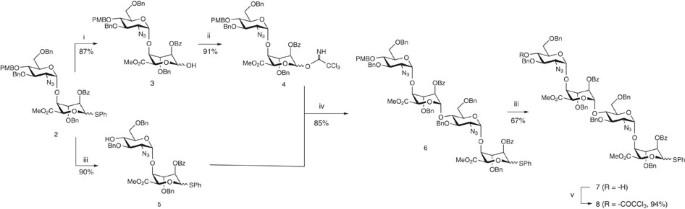Figure 2: Synthesis of core tetrasaccharide donor/acceptor modules. (i) NBS, acetone. (ii) CCl3CN, DBU, DCM. (iii) CAN, CH3CN/H2O. (iv) TMSOTf, DCM. (v) CCl3COCl, pyridine, DCM. Figure 2: Synthesis of core tetrasaccharide donor/acceptor modules. (i) NBS, acetone. (ii) CCl 3 CN, DBU, DCM. (iii) CAN, CH 3 CN/H 2 O. (iv) TMSOTf, DCM. (v) CCl 3 COCl, pyridine, DCM. Full size image Synthesis of tetrasaccharide 6 was similarly efficient whether thioglycoside acceptor α- 5 or β- 5 was employed, providing access to either tetrasaccharide α- 7 or β- 7 , respectively, both of which can function in the subsequent iterative homologations to effect the same α-selective glycosylations of the desired oligosaccharide acceptor. These tetrasaccharides can readily be accessed on hundreds of milligram to multigram scale. Notably, and further enhancing the overall synthetic efficiency, although 7 has both acceptor (4-OH) and donor (1-SPh) functionality, this material could be directly glycosylated at the reducing terminus without the need for protection at O4. The installation of the required LAT was thus effected using a dibenzylated glycerol unit, designed for its ultimate deprotection to the required diol concomitant with the penultimate debenzylation of the protected heparin oligosaccharide. Hence, 7 was glycosylated with ( S )-2,3-dibenzyloxy propanol affording the reducing end-modified tetrasaccharide acceptor 9 (see Supplementary Figs S32–S36 ) directly, with the non-reducing terminus already in place as an acceptor for the first tetrasaccharide homologation ( Fig. 3 ). 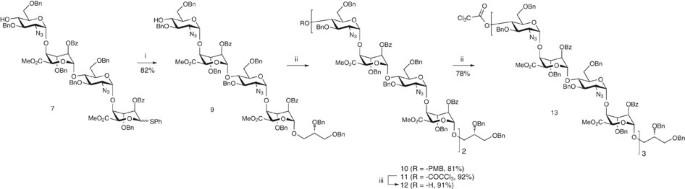Figure 3: Iterative [4+4+4] dodecasaccharide synthesis. (i) (S)-2,3-bis(benzyloxy)propanol, NIS, AgOTf (cat.), DCM. (ii)6or8, NIS, AgOTf (cat.), DCM. (iii) MeOH/pyridine (5:2). Figure 3: Iterative [4+4+4] dodecasaccharide synthesis. (i) ( S )-2,3-bis(benzyloxy)propanol, NIS, AgOTf (cat. ), DCM. (ii) 6 or 8 , NIS, AgOTf (cat. ), DCM. (iii) MeOH/pyridine (5:2). Full size image Coupling of acceptor 9 and tetrasaccharide donors 6 or 8 , hence, generated the octasaccharides 10 (see SupplementaryFigs S37–S39 ) and 11 (see Supplementary Figs S40–S44 ), respectively, with complete α-anomeric selectivity. This now further establishes that the iduronate donor-terminated tetrasaccharides can function as efficient oligosaccharide homologation building blocks using longer acceptors (a previous GlcN-GlcA-GlcN-IdoA tetrasaccharide had been shown to be effective as a donor for monosaccharide acceptors) [24] and compliments such a capability exploited using GlcN donor systems [24] , [44] . This also thereby underpins a capability to now access other long [GlcN-IdoA] n -based sequences using such an accelerated iterative strategy. Synthesis of oligosaccharide via [4+4+4] two-cycle iteration During the deprotection of O4 of octasaccharide 10 , it was found that the ceric ammonium nitrate mediated p -methoxybenzyl removal gave a mixture of products, although the TCA group of analogue 11 could be removed in excellent yield using novel mild conditions. Combined with the higher glycosylation yields obtained, this led to selection of the O4-TCA tetrasaccharide 8 for further iterations. Deprotection of octasaccharide 11 provided acceptor octasaccharide 12 (see Supplementary Figs S45–S49 ) as a substrate, enabling a second cycle of iterative coupling with donor module 8 , providing thereby protected dodecasaccharide 13 (see Supplementary Figs S50–S54 ) and completing the efficient and rapid two-cycle iteration. The overall four-step yield from tetrasaccharide 7 to protected dodecasaccharide 13 was 54%, yielding around 300 mg of this oligosaccharide, a significant scale for such rapid dodecasaccharide assembly. From protected dodecasaccharide 13 , concurrent saponification, O -sulphation, debenzylation/azide reduction and finally N -sulphation provided the fully deprotected and regiospecifically sulphated dodecasaccharide 14 (see Supplementary Figs S59–S64 ) bearing the free 1,2-diol LAT unit at the reducing terminus ( Fig. 4 ). 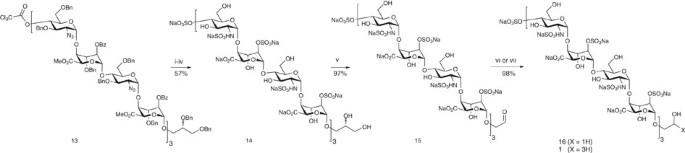Figure 4: Dodecasaccharide deprotections and end labelling. (i) LiOH, tetrahydrofuran (THF)/MeOH/H2O, 74%. (ii) Py.SO3complex, pyridine, 80%. (iii) H2, Pd(OH)2/C, MeOH/THF/H2O 2:1:1, 96%. (iv) Py.SO3complex, NaHCO3, H2O, 100%. (v) NaIO4, H2O. (vi) NaBH4, H2O. (vii) NaB3H4, H2O. Figure 4: Dodecasaccharide deprotections and end labelling. (i) LiOH, tetrahydrofuran (THF)/MeOH/H 2 O, 74%. (ii) Py.SO 3 complex, pyridine, 80%. (iii) H 2 , Pd(OH) 2 /C, MeOH/THF/H 2 O 2:1:1, 96%. (iv) Py.SO 3 complex, NaHCO 3 , H 2 O, 100%. (v) NaIO 4 , H 2 O. (vi) NaBH 4 , H 2 O. (vii) NaB 3 H 4 , H 2 O. Full size image Nuclear magnetic resonance provides unambiguous definition of the complete N -sulphation, evidenced by the clear difference in shift of the H-2 protons on converting the 2-amino to 2-NS functionality ( Fig. 5 ). Differentiation of the NS of the non-reducing terminal glucosamine 2-NS is evident (the only ring with O4-S) and confirmed by clear correlation spectroscopy correlations (see Supplementary Fig. S60 ). The clear resolution of signals for the reducing terminal iduronate is clear, and on oxidative cleavage the spectrum for the RAT-terminated dodecasaccharide shows a clear set of two doublets (1.3:1) for the RAT methylene. These are not mutually coupled and the non-equivalent integration would also be consistent with these arising from acetal formation, transiently retaining the LAT aldehyde in a seven-membered ring hemiacetal. This is also consistent with changes in the shifts of H5 and H2 of the reducing terminal iduronate. In addition, the H-5 of ring A is well separated and the small coupling constant for those protons, also evident for the other overlapping H5 protons, shows that these long sulphated oligosaccharides do sit largely in the ido 1 C 4 conformation. 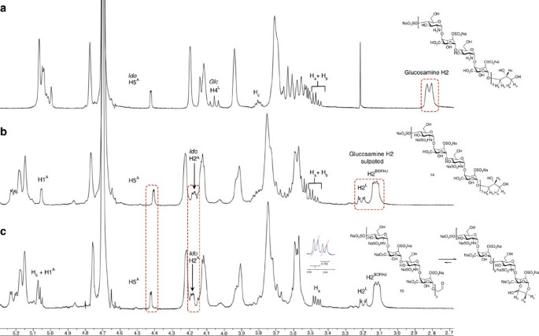Figure 5: Nuclear magnetic resonance confirmation of dodecasaccharideN-sulphation and comparisons of diol LAT and oxidatively cleave RAT. (a) Intermediate amino containing dodecasaccharide. (b)N-sulphated dodecasaccharide. (c) Oxidatively cleaved RAT-terminated oligosaccharide. Figure 5: Nuclear magnetic resonance confirmation of dodecasaccharide N -sulphation and comparisons of diol LAT and oxidatively cleave RAT. ( a ) Intermediate amino containing dodecasaccharide. ( b ) N -sulphated dodecasaccharide. ( c ) Oxidatively cleaved RAT-terminated oligosaccharide. Full size image Oxidative cleavage was effected in near-quantitative yield with sodium periodate, unveiling the target-reducing end aldehyde in the form of reactive conjugate, 15 (see Supplementary Figs S65–S67 ). To introduce the tritium label, 15 was then treated with NaB 3 H 4 under basic conditions at 45 °C (following cold-label method evaluations on a disaccharide model and the unlabelled reduction of 15 to 16 (see Supplementary Figs S68–S70 )). After ensuring the reaction was complete by addition of excess NaBH 4 and quenching, the sample was desalted on Sephadex G-25 to remove excess reducing agent. Radiolabelled 1 was then further purified by size-exclusion chromatography ( Fig. 6 ) and was eluted from the column in good accordance with an established de-6- O -sulphated dodecasaccharide heparin standard. The specific activity of 1 was determined to be 5.5 × 10 6 c.p.m. mg −1 of oligosaccharide, suitable for the required in vivo evaluations. 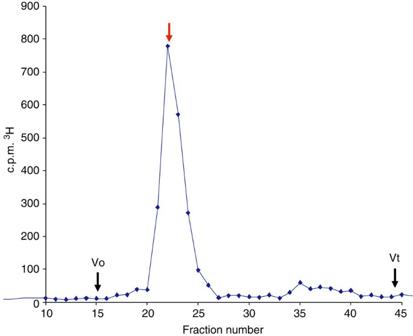Figure 6: HPLC size-exclusion chromatogram of 1 on Superdex. To confirm the oligomer size of3H-1HPLC size-exclusion chromatography on Superdex 75 indicated the3H-1elutes (red arrow) at position identical to de-6-O-sulphated dodecasaccharide heparin standard. Vo, excluded volume; Vt, total column volume. Figure 6: HPLC size-exclusion chromatogram of 1 on Superdex. To confirm the oligomer size of 3 H- 1 HPLC size-exclusion chromatography on Superdex 75 indicated the 3 H- 1 elutes (red arrow) at position identical to de-6- O -sulphated dodecasaccharide heparin standard. Vo, excluded volume; Vt, total column volume. Full size image Applications of radiolabelled heparin dodecasaccharide 1 Radiolabelled heparin-mimetic 1 was thus employed to determine its in vivo clearance and tissue distribution in mice (the biological efficacy of the OMe analogue of which we had previously established in vitro ) [52] . The mice were dosed subcutaneously (s.c.) with 20, 40 and 80 mg kg −1 of oligosaccharide spiked with 140,000 c.p.m. of 3 H-12-mer 1 as a radiotracer. Tissue concentrations were determined from the level of radiolabelled oligosaccharide in tissue samples of known mass during a 16-h period ( Fig. 7 ). A maximum plasma concentration of 18 μg ml −1 was observed 15 min after dosing mice with 20 mg kg −1 of oligosaccharide ( Fig. 6a ). When dosed with 40 or 80 mg kg −1 , maximum plasma concentrations of 44.8 and 84.0 μg ml −1 , respectively, were observed after 60 min ( Fig. 6b ). Critically, these data demonstrate that the plasma concentration of oligosaccharide in vivo was sufficient to inhibit the biological activity of FGF2 based on in vitro data [52] . 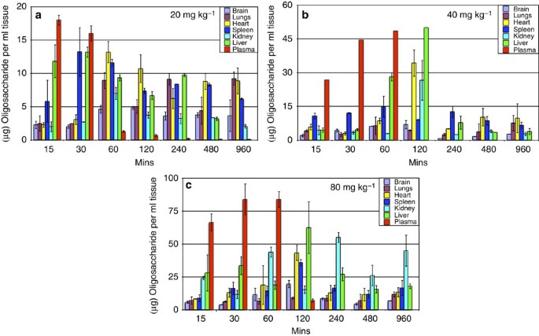Figure 7: Tissue localisation of 1. Mice (two) were injected with 20 (a), 40 (b) or 80 mg kg−1(c) of1. Tissue quantities are presolublization. Error bars represent the s.e.m. of c.p.m. converted to oligo weight using specific activity. Figure 7: Tissue localisation of 1. Mice (two) were injected with 20 ( a ), 40 ( b ) or 80 mg kg −1 ( c ) of 1 . Tissue quantities are presolublization. Error bars represent the s.e.m. of c.p.m. converted to oligo weight using specific activity. Full size image All tissues, except lungs, showed a time-dependent accumulation of 1 at all doses, and the maximum concentrations increased with a higher initial dose ( Fig. 6 ). The highest concentration of 1 was detected in tissues when mice were treated with 80 mg kg −1 . In addition, all tissues, except the liver, attained maximal levels of 1 by 120 min. The tissue distribution data described here show that at 40 and 80 mg kg −1 , biologically active concentrations [52] were achieved in the liver, lungs and spleen within a 2-h period. The half-life of oligosaccharides in mice was estimated to be ~2 h. As murine clearance is so rapid, this result is particularly encouraging for the development of oligosaccharide therapeutics. From the results shown in Fig. 6 , there is good evidence for sustained plasma concentrations of 1 up to around 1 h at the two higher dose levels and that the oligosaccharide is well retained in the plasma at these concentrations. At lower doses, there is a more even distribution among the examined tissues, suggesting that higher doses would be needed to sustain sufficient oligosaccharide concentration in plasma. To assess the metabolic stability of 1 in vivo , we extracted and purified 3 H-12-mer 1 from mouse kidney after a 4-h treatment, to determine the extent of any degradation or metabolism. The majority of the material eluted in a single peak of 3,500 Da, which corresponds to a mass of dodecasaccharide 1 ( Fig. 8 ). 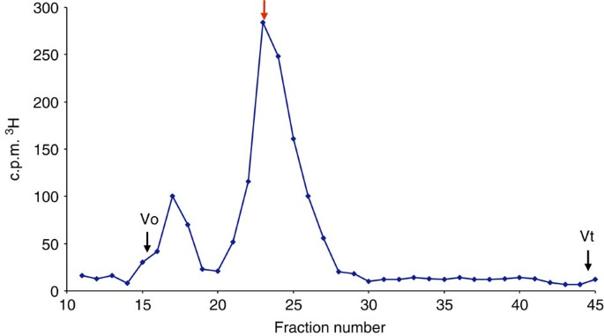Figure 8: HPLC SEC of 1 injected s.c. into mice and then extracted and purified from kidneys 4 h after injection. Radiolabelled oligosaccharide1was injected s.c. into mice and then extracted and purified from kidneys 4 h after injection (seeMethods). Radiolabelled oligosaccharide1was subjected to HPLC chromatography on a Superdex 75 size-exclusion column. Red arrow shows elution of3H-1(seeFig. 5). Vo, excluded volume; Vt, total column volume. Figure 8: HPLC SEC of 1 injected s.c. into mice and then extracted and purified from kidneys 4 h after injection. Radiolabelled oligosaccharide 1 was injected s.c. into mice and then extracted and purified from kidneys 4 h after injection (see Methods ). Radiolabelled oligosaccharide 1 was subjected to HPLC chromatography on a Superdex 75 size-exclusion column. Red arrow shows elution of 3 H- 1 (see Fig. 5 ). Vo, excluded volume; Vt, total column volume. Full size image This [4+4+4] iterative oligosaccharide approach thus provides an efficient two-cycle synthesis of a structurally defined HS dodecasaccharide, illustrating that iduronate donor tetrasaccharides function as effective and selective glycosyl donors with extended saccharide acceptors. The reduction here in the number of synthetic steps taken to assemble these longer heparanoids significantly enhances their accessibility, and the inclusion of the end label via glycosylation (avoiding O4 protection) to directly afford an end-tagged tetrasaccharide acceptor also adds to the abbreviation of the synthetic route. Notably, homologation here using 4-mer and 8-mer acceptors with this longer donor is shown to perform with an efficiency that remains high, even for a [4+8] coupling. The efficiency of this tetrasaccharide-iteration-based synthetic route also facilities the viability of new opportunities for sequence versatility and applications to other diverse conjugation targets. The synthesis and inclusion of the LAT described here offers a unique strategy for discrete end labelling of this heparin-like structure, such that the label will not interfere with the ligand-binding potential of the molecule, and the small structural change would be anticipated to minimize effects on pharmacokinetics. The end-terminal latent tag offers generality for incorporation into other heparanoids. Utility of this end group for radiolabelling provides the first example of using a structurally defined heparin-like dodecasaccharide to quantify in vivo tissue distribution and metabolic stability. Conventional pharmacological development of heparin has relied on its anticoagulant properties that can be measured in patients using universally available tests of the clotting cascade. However, the lack of anticoagulant activity of structurally defined synthetic HS oligosaccharides, although important for non-anticoagulant drugs, also presents the problem of how to measure the pharmacokinetics and metabolism of such novel synthetic heparin-like oligosaccharides in vivo . Here we report for the first time a novel solution to this problem that should greatly assist the preclinical and clinical development of potential oligosaccharide therapeutics. In this dodecasaccharide case, this study has shown that the dodecasaccharide has good in vivo stability, and strongly indicates that oligosaccharide drugs of this type have a high prospect of effective dose distribution and stability on therapeutically valid timescales. Synthesis of dodecasaccharide 12 Octasaccharide 11 (346 mg, 0.10 mmol) was dissolved in a mixture of MeOH/pyridine (5 ml per 2 ml) and heated to 50 °C for 4 h. The solvents were evaporated and coevaporated with toluene (2 × 20 ml). The crude product was purified using flash column chromatography (EtOAc/hexane 1:2 and 3:5). This yielded 12 (300 mg, 91%) as a white foam, along with recovered starting material (20 mg, 5%). R f 0.10 (EtOAc/hexane 1:2). [α] D 20 =+9.8 ( c =0.32, CH 2 Cl 2 ). Mass spectrometry (MS) matrix-assisted laser desorption/ionization–time of flight: m/z : calcd for C 181 H 184 N 12 NaO 47 [ M +Na] + : 3300.2; found: 3300.2. Elemental analysis calcd (%) for C 181 H 184 N 12 O 47 : C 66.29, H 5.66, N 5.13; found C 66.57,H 5.98, N 4.96 (see Supplementary Methods for further characterization data). Synthesis of dodecasaccharide 13 Acceptor 12 (252 mg, 0.077 mmol) and donor 8 (175 mg, 0.100 mmol) were dissolved in dry dichloromethane (DCM) (4 ml) under N 2 . Freshly activated 4 Å powdered molecular sieves (222 mg) were added and the solution cooled to 0 °C in an ice bath. After 10 min NIS (47 mg, 0.21 mmol) was added, and after another 10 min AgOTf (catalytic amount) was added. The suspension changed colour from pale yellow to deep red and was stirred for a further 35 min. The reaction was quenched into a separating funnel containing a mixture of DCM (50 ml), saturated aqueous NaHCO 3 (50 ml) and Na 2 S 2 O 3 (5 ml, 10% aqueous). After shaking until the iodine colour was removed, the suspension was filtered through a short pad of Celite washing with water and DCM. The layers were separated and the aqueous layer extracted with DCM (10 ml). The organic layers were combined, dried (MgSO 4 ) and the solvent removed in vacuo . The crude product was purified by silica gel flash column chromatography (EtOAc/hexane 7:13) to yield 13 (295 mg, 78%) as a white foam (recovered acceptor (37 mg, 15%)). [α] D 20 =+18.1 ( c =0.68, CH 2 Cl 2 ). MS matrix-assisted laser desorption/ionization–time of flight: m/z : calcd for C 265 H 265 Cl 3 N 18 NaO 70 [ M +Na] + : 4946.7; found: 4946.6. Elemental analysis calcd (%) for C 265 H 265 Cl 3 N 18 O 70 : C 64.58, H 5.42,N 5.12; found C 63.91, H 5.41, N 5.06 (see Supplementary Methods for further characterization data). Synthesis of dodecasaccharide sodium salt 14 Saponifications . Dodecasaccharide 13 (257 mg, 0.052 mmol) was dissolved in tetrahydrofuran (5 ml) and MeOH (1.5 ml), and then cooled to 0 °C in an ice bath. Then, LiOH.H 2 O (55 mg, 1.30 mmol) dissolved in 1 ml water was added dropwise over 10 min. The solution was stirred for 5 h at 0 °C, and then at room temperature for another 19 h. The solution was then extracted with EtOAc (2 × 50 ml) and HCl (0.2 M, 40 ml), dried (MgSO 4 ), filtered and evaporated. The crude product was purified using flash column chromatography (DCM/MeOH 30:1). This yielded the carboxylic acid dodecasaccharide intermediate product A (174 mg, 74%) as a white solid. R f 0.18 (DCM/MeOH 20:1), then used directly in the next step. Sulphation of hydroxyls The dodecasaccharide intermediate A (170 mg, 0.042 mmol) was dissolved in dry pyridine (5 ml), pyridine sulphur trioxide complex (140 mg, 0.88 mmol) added and then heated to 50 °C in an oil bath for 8 h. The solution was stirred at room temperature for another 12 h. The reaction was quenched with MeOH and then evaporated. The crude product was redissolved in MeOH/DCM (10 ml/5 ml), stirred with Amberlite IR-120 Na + resin (1.3 g) for 8 h, filtered, resin washed with MeOH (2 × 5 ml) and the filtrate evaporated. This residue was then purified using flash column chromatography (DCM/MeOH 20:1). This yielded 2- O -sulphated dodecasaccharide intermediate B ( 160 mg, 80%) as a white solid. Hydrogenolysis of benzyls and azides The IdoA2S benzylated 2-azido-containing dodecasaccharide intermediate B (132 mg, 0.027 mmol) was dissolved in a mixture of MeOH/tetrahydrofuran (4 ml/2 ml), and NaHCO 3 (14 mg, 0.165 mmol) dissolved in 2 ml of water was added, atmosphere exchanged for nitrogen and Pd(OH) 2 /C (120 mg, 10–20%) added, and again flushed with nitrogen. The nitrogen balloon was replaced with a hydrogen balloon and atmosphere replaced with hydrogen. The reaction was heated to 40 °C in an oil bath for 48 h with vigorous stirring. The product mixture was filtered through Celite, washed with MeOH/water (3 × 3 ml) and water (3 × 3 ml). The combined filtrate was then evaporated to give dodecasaccharide amine intermediate C (78 mg, 96%) as a glassy solid (see Supplementary Methods ). Sulphation of amines The dodecasaccharide amine (65 mg, 0.022 mmol) was dissolved in water (4 ml), NaHCO 3 (108 mg, 1.29 mmol) and pyridine sulphur trioxide complex (97 mg, 0.61 mmol) was added with vigorous stirring. This procedure was repeated after 1.30, 3.30, 5.30, 17.30 and 19.30 h (NaHCO 3 : 109, 121, 113, 110 and 110 mg; Py.SO 3 : 92, 88, 111, 100 and 70 mg). After 24 h, the mixture was evaporated. The crude containing Na 2 SO 4 salts was redissolved in minimum amount of water and purified by passage through a Sephadex G-25 column (40 ml) by eluting with water. The fractions containing oligosaccharide were pooled and evaporated to yield 14 ( 78 mg, 100%) of as a glassy solid. High-resolution MS (Fourier transform MS): m/z : calcd for C 75 H 111 N 6 Na 4 O 102 S 13 [ M -15Na+8H] −7 : 462.4234; found: 462.4244 (see Supplementary Methods for structures of intermediates A , B and C , and further characterization data for B , C and 14, and Supplementary Figs 56–59 for spectra of A–C ). Synthesis of dodecasaccharide aldehyde 15 The dodecasaccharide 14 (61 mg, 0.017 mmol) was dissolved in water (1 ml) and sodium periodate (3.9 mg, 0.018 mmol) was added and stirred for 6 h. The crude was purified by passage through a Sephadex G-25 column by eluting with water. The fractions containing oligosaccharide were pooled and evaporated to yield 58 mg (97%) of 15 as a glassy solid (see Supplementary Methods for characterization data). Synthesis of 3 H-labelled dodecasaccharide 1 Three micrograms of 3 H-labelled sodium borohydride (1 mCi) was reacted with 1.2 mg of aldehyde-bearing dodecasaccharide 15 in 20 μl of 50 mM NaOH in a sealed reinforced glass Reacti-Vial at 45 °C for 2 h. To ensure that all aldehyde was reduced, an excess of unlabelled 1 M sodium borohydride was then added and sample incubated for a further 2 h at 45 °C. Reaction was halted by the addition of 5 μl of 1 M sulphuric acid. Tritium-labelled oligosaccharide was then desalted on PD-10 (G-25) column that was pre-equilibrated with water and 0.5 ml fractions were collected. Labelled oligosaccharide 1 , which eluted in fractions 10–14, was collected and freeze-dried. To confirm the size of radiolabelled material, the 3 H-dodecasaccharide 1 was subjected to HPLC size-exclusion chromatography on an Agilent 1200 HPLC system. The sample was run on a Superdex 75 column (10 mm × 300 mm; GE Healthcare) in PBS at 0.5 ml min −1 . Aliquots from 0.5 ml fractions were taken, mixed with 2 ml of Hisafe scintillation fluid (Perkin-Elmer) and 3 H level was counted on a Wallac 1400 scintillation counter. An unlabelled de-6- O -sulphated heparin dodecasaccharide (Iduron), which is approximately the same size as synthetic dodecasaccharide 1 , was used to calibrate the column and was monitored at 232 nm by an in-line ultraviolet detector. Fractions containing 3 H-dodecasaccharide 1 were collected, desalted, freeze-dried and weighed. Specific activity was determined as 5.5 × 10 6 c.p.m. mg −1 of oligosaccharide. Pharmacokinetic study of 3 H-labelled dodecasaccharide 1 in mice 3 H-Labelled dodecasaccharide 1 was administered to SCID- bg female mice s.c. as a single dose at 20, 40 and 80 mg kg −1 and animals were culled at 0.25, 0.5, 1, 2, 4, 8 and 16 h after dosing. Two animals per each treatment group were used. At the time of culling, blood was collected by cardiac puncture. The brain, kidney, liver, spleen, heart and lungs were removed and their weight was measured. Samples were incubated overnight at 60 °C in 4 ml of Soluene 350 (Perkin-Elmer). Aliquots of 500 μl of the resultant tissue solution were taken for scintillation counting. Plasma was obtained by centrifuging mouse blood at 1,500 r.p.m. in a bench top Eppendorf microcentrifuge and collecting the supernatant. Plasma (100 μl) was added to 2 ml of scintillation fluid and 3 H levels were determined by scintillation counting. Concentration of oligosaccharide in plasma and tissues was derived from the specific activity of the radiolabel (see above). Extraction and purification of 3 H-12-mer dodecasaccharide 1 from mouse kidney To assess the stability of 3 H-dodecasaccharide 1 in vivo , one animal was dosed with 1 at 20 mg kg −1 for 4 h, and HS was extracted from mouse kidney post mortem using a routine method for HS extraction [59] . The kidneys were dissolved for 16 h at 60 °C in 4 M guanidine HCl/8 M urea/1% Triton in 50 mM Tris, pH 8.0. The extract was diluted 1:100 with water and applied to a 1 ml DEAE-Sephacel (Sigma) ion exchange column pre-equilibrated with PBS. The resin was then washed with 5 ml of 100 mM phosphate buffer with 0.25 M NaCl to remove hyaluronan and non-GAG material. The oligosaccharide was eluted with 1 M NaCl in phosphate buffer, concentrated to 1 ml and subjected to size-exclusion HPLC chromatography on a Superdex 75 column in PBS. Fractions (0.5 ml) were collected and counted. How to cite this article: Hansen, S. U. et al . Tetrasaccharide iteration synthesis of a heparin-like dodecasaccharide and radiolabelling for in vivo tissue distribution studies. Nat. Commun. 4:2016 doi: 10.1038/ncomms3016 (2013).